Electrostatic charging of jumping droplets With the broad interest in and development of superhydrophobic surfaces for self-cleaning, condensation heat transfer enhancement and anti-icing applications, more detailed insights on droplet interactions on these surfaces have emerged. Specifically, when two droplets coalesce, they can spontaneously jump away from a superhydrophobic surface due to the release of excess surface energy. Here we show that jumping droplets gain a net positive charge that causes them to repel each other mid-flight. We used electric fields to quantify the charge on the droplets and identified the mechanism for the charge accumulation, which is associated with the formation of the electric double layer at the droplet–surface interface. The observation of droplet charge accumulation provides insight into jumping droplet physics as well as processes involving charged liquid droplets. Furthermore, this work is a starting point for more advanced approaches for enhancing jumping droplet surface performance by using external electric fields to control droplet jumping. Exactly 100 years ago in 1913, Robert A. Millikan [1] analysed the motion of electrified droplets in a uniform electric field to quantify the charge of an electron. Since then, researchers have studied the mechanism of charge accumulation on atomized droplets [2] , sessile droplets [3] , [4] , [5] and the hydrophobic coatings beneath them [6] , [7] , [8] , [9] , sometimes using a modification of Millikan’s approach [5] . Recently, with the broad interest in and development of superhydrophobic surfaces [10] , [11] for a variety of applications including self-cleaning [12] , condensation heat transfer enhancement [13] , [14] , [15] , [16] , [17] , [18] , [19] , [20] , [21] , thermal diodes [22] , [23] and anti-icing [24] , [25] , [26] , [27] , more detailed insights on droplet interactions on these surfaces have emerged. Specifically, when two or more small droplets (≈10–100 μm) coalesce, they can spontaneously jump away from a superhydrophobic surface due to the release of excess surface energy [28] , which promises enhanced system performance by passively shedding water droplets [13] , [15] . To date, researchers have focused on creating superhydrophobic surfaces showing rapid droplet removal [29] , [30] , [31] , [32] , [33] , [34] , [35] , [36] , [37] and experimentally analysing [14] , [16] , [30] , [38] and modelling [39] , [40] the merging and jumping behaviour before and immediately after coalescence. However, aspects related to the droplet charging during the formation, growth and jumping of droplets have not been identified. Here, we show that jumping droplets gain a net positive charge that causes them to repel each other mid-flight. In a modified experiment inspired by that of Millikan [1] , we use uniform electric fields to quantify the charge on the droplets. By studying a variety of hydrophobic coatings and structure length scales, we show that the charge is dependent on the surface area of the departing droplets and the hydrophobic coating beneath them. Accordingly, we explain the mechanism for the charge accumulation, which is associated with the formation of the electric double layer at the droplet–coating interface, and subsequent charge separation during droplet jumping. Our results demonstrate the important role of surface charge interactions on jumping droplet dynamics and also provide insight into jumping droplet physics. This work is also a starting point for more advanced approaches for enhancing jumping droplet surface performance. For example, an external electric field can control the jumping efficiency to enhance condensation heat transfer, anti-icing and self-cleaning performance. In addition, the charge separation phenomenon promises an advantageous metrology to characterize the zeta potential of hydrophobic coatings on large-scale superhydrophobic surfaces. Furthermore, the identified electric double layer charge separation [41] and droplet charging can be used for atmospheric electric power generation. Jumping droplet interactions To characterize droplet–droplet interactions on a well-defined surface, we first investigated the jumping droplet behaviour of copper (Cu) tubes coated with functionalized copper oxide (CuO) nanostructures ( Fig. 1a , see Methods) by condensing water vapour on the surface and observing droplet jumping. Hydrophobic functionalization was obtained by depositing a fluorinated silane (trichloro(1H, 1H, 2H, 2H-perfluorooctyl)silane, Sigma-Aldrich) in the vapour phase (see Methods). This self-assembled silane coating (hereafter labelled ‘TFTS’) had a typical advancing angle of θ a ≈120° when measured on a smooth reference surface and typical advancing/receding angles of θ a / θ r ≈171/167±3° when measured on the nanostructured CuO surface. To observe droplet jumping, the CuO tubes were tested in a controlled condensation chamber (see Methods). Before performing the experiments, the water for the vapour supply was vigorously boiled and the test chamber was evacuated to a pressure P <0.5±0.025 Pa to eliminate non-condensable gases. Throughout the experiments, the chamber pressure and temperature were continuously monitored to ensure saturated conditions. The temperature of the tube was independently controlled via a cooling loop (see Methods). 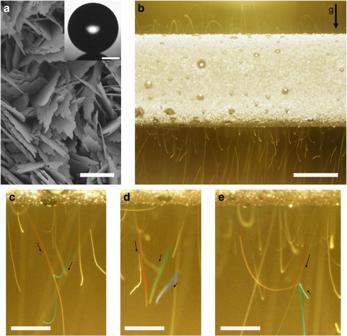Figure 1: Nanostructure characterization and jumping droplet interactions. (a) Field emission scanning electron micrograph of a 10-min-oxidized CuO surface. Scale bar, 500 nm. The sharp, knife-like CuO structures have characteristic heights,h≈1 μm, solid fraction,φ≈0.023 and roughness factor,r≈10. (inset: water droplet contact advancing angle on the nanostructured superhydrophobic surface,θa=169±3°. Scale bar, 20 μm) (b) Long exposure time image (50 ms) of jumping-droplet condensation on a nanostructured CuO tube showing droplet–droplet interactions and droplet return to the bottom surface against gravity (seeSupplementary Movie 1). Scale bar is 3 mm. (c–e) Long exposure time (50 ms) false-colour images of droplet–droplet repulsive interactions (seeSupplementary Movies 2, 3 and 4). Scale bar, 1 mm. Chamber vapour pressurePv=2,700±68 Pa,S≈1.06. The tube sample (outer diameterDOD=6.35 mm, inner diameterDID=3.56 mm and lengthL=131 mm) was cooled via chilled water flowing inside the tube at 5±0.25 l min−1, see Methods). Figure 1: Nanostructure characterization and jumping droplet interactions. ( a ) Field emission scanning electron micrograph of a 10-min-oxidized CuO surface. Scale bar, 500 nm. The sharp, knife-like CuO structures have characteristic heights, h ≈1 μm, solid fraction, φ ≈0.023 and roughness factor, r ≈10. (inset: water droplet contact advancing angle on the nanostructured superhydrophobic surface, θ a =169±3°. Scale bar, 20 μm) ( b ) Long exposure time image (50 ms) of jumping-droplet condensation on a nanostructured CuO tube showing droplet–droplet interactions and droplet return to the bottom surface against gravity (see Supplementary Movie 1 ). Scale bar is 3 mm. ( c – e ) Long exposure time (50 ms) false-colour images of droplet–droplet repulsive interactions (see Supplementary Movies 2, 3 and 4 ). Scale bar, 1 mm. Chamber vapour pressure P v =2,700±68 Pa, S ≈1.06. The tube sample (outer diameter D OD =6.35 mm, inner diameter D ID =3.56 mm and length L =131 mm) was cooled via chilled water flowing inside the tube at 5±0.25 l min −1 , see Methods). Full size image Figure 1b shows a long exposure time image (50 ms) taken during steady-state condensation on the CuO tube (see Supplementary Movie 1 ), where the white streaks are the trajectories of the jumping droplets. The CuO surface showed very efficient droplet removal via the jumping mechanism, with numerous microscale droplets departing from the surface. Figure 1b also shows significant droplet–droplet interactions after droplets departed from the surface, as seen by the changes in the droplet trajectories. Figure 1c–e highlights that when droplets approach one another, they tend to repel each other and do not coalesce (see Supplementary Movies 2, 3 and 4 ), an unexpected observation if the droplets were neutral [42] . Instead, the mid-flight repulsion indicates that droplets may carry electric charge. Furthermore, the uniform repulsive interaction of droplets shows that the charge polarity, that is, positive or negative, must be identical for all jumping droplets. To further study the charging hypothesis and elucidate the charge polarity, we modified the experimental setup to include an electrode ( Fig. 2a , see Methods, and Supplementary Fig. S4 ). The electrode was a 350-μm-diameter copper wire, and was connected to a 600-V direct current (DC) power supply (N5752A, Agilent Technologies) with the opposite terminal connected to the grounded tube sample. The electrode was placed beneath the superhydrophobic surface to allow interactions between the electrode and droplets passing under the influence of gravity. With an applied constant electrical bias (Δ V ), an electric field between the electrode and grounded tube was established, creating droplet motion towards or away from the electrode depending on the polarity of the bias (negative or positive). 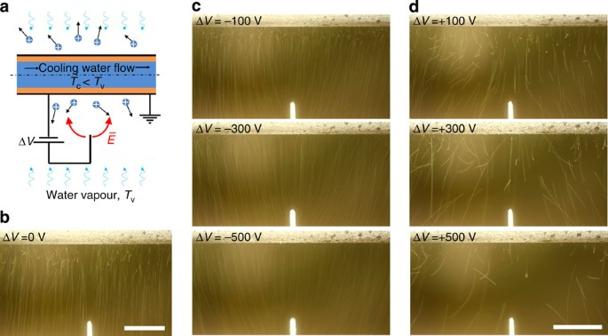Figure 2: Droplet interactions with an electric field. (a) Schematic showing experimental setup. A copper wire electrode was placed ≈5 mm beneath the tube and voltage biased relative to the tube sample (ΔV). The voltage potential difference created an electrostatic field (Ē) allowing for the charged droplet interactions with the field to be observed. Long exposure time images (50 ms) of jumping-droplet condensation with (b) no electric field, (c) negative electric field (electrode is negative, tube is grounded) and (d) positive electric field (electrode is positive, tube is grounded). Scale bar, 3 mm. Under zero bias (ΔV=0), droplets jump from the surface and travel downwards past the electrode. When the electrode was biased with a negative voltage (ΔV=−100, −300 and −500 V), attraction between the departing droplets and electrode was observed (seeSupplementary Movies 4, 6 and 7). When the electrode was biased with a positive voltage (ΔV=+100, +300 and +500 V), repulsion between the droplets and electrode was observed (seeSupplementary Movies 8, 9 and 10). The results are consistent with the droplets being positively charged (chamber vapour pressurePv=2,700±68 Pa,S≈1.04). Figure 2b shows a long exposure time image (50 ms) of droplet motion in the presence of the electrode with Δ V =0. As expected, droplet–droplet interactions were observed close to the tube sample, whereas no electrode–droplet interactions were apparent due to the neutrality of the electrode. However, when a negative bias was applied to the electrode (Δ V =−100, −300, −500 V), significant droplet–electrode attraction was observed ( Fig. 2c , see Supplementary Movies 5–7 ). To eliminate the possibility of induced electrical effects, that is, droplet motion due to dielectrophoresis, we reversed the polarity of the electrode (Δ V =+100, +300, +500 V) and saw a significant droplet–electrode repulsion ( Fig. 2d , see Supplementary Movies 8–10 ). The repulsion and attraction observed under positive and negative electrode bias, respectively, indicates that dielectrophoresis was not the cause of droplet–electrode interaction and that all of the droplets were positively charged after jumping from the surface. Although the magnitude of the droplet charge can be calculated from these electrode experiments, potential charging of the hydrophobic surface coating may arise [6] , [9] , altering the voltage bias so that the magnitude of the electric field is difficult to determine. It is also important to note that, although charging may occur from the tube substrate beneath the nanostructure via flow electrification [43] , droplet charging was found to be independent of the cooling water flow rate, thus eliminating this possibility. Figure 2: Droplet interactions with an electric field. ( a ) Schematic showing experimental setup. A copper wire electrode was placed ≈5 mm beneath the tube and voltage biased relative to the tube sample (Δ V ). The voltage potential difference created an electrostatic field ( Ē ) allowing for the charged droplet interactions with the field to be observed. Long exposure time images (50 ms) of jumping-droplet condensation with ( b ) no electric field, ( c ) negative electric field (electrode is negative, tube is grounded) and ( d ) positive electric field (electrode is positive, tube is grounded). Scale bar, 3 mm. Under zero bias (Δ V =0), droplets jump from the surface and travel downwards past the electrode. When the electrode was biased with a negative voltage (Δ V =−100, −300 and −500 V), attraction between the departing droplets and electrode was observed (see Supplementary Movies 4, 6 and 7 ). When the electrode was biased with a positive voltage (Δ V =+100, +300 and +500 V), repulsion between the droplets and electrode was observed (see Supplementary Movies 8, 9 and 10 ). The results are consistent with the droplets being positively charged (chamber vapour pressure P v =2,700±68 Pa, S ≈1.04). Full size image Droplet charge measurement To better control the electric field, we adapted an approach similar to that of Millikan [1] , whereby external parallel plates were used to create a uniform field. 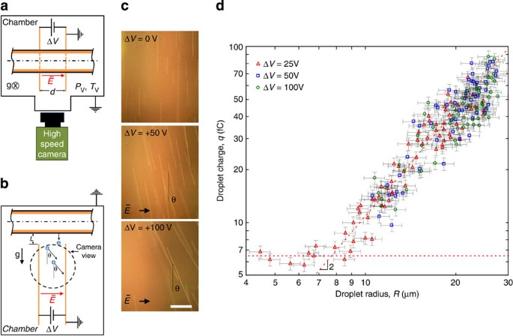Figure 3: Experimental setup and images of droplet deflection. Schematic showing (a) top view and (b) side view of the experimental setup used to measure individual droplet charge. Two 10 × 20 cm polished parallel copper plates were placedL=10±0.5 mm beneath the tube and spacedd=19±0.05 mm apart. The plates were voltage biased relative to one another to create a uniform electric field. High-speed imaging of droplet motion inside the constant electric field beneath the tube sample allowed for the quantification of individual droplet charge for fields ofĒ=ΔV/d=1.31, 2.63 and 5.26 kV m−1. (c) Long exposure time images (33 ms) of droplet motion between the parallel plates at field strengths ofĒ=0, 2.63 and 5.26 kV/m (seeSupplementary Movies 11, 12 and 13). Left side of the images is the positive plate and right side is the grounded plate. Scale bar, 4 mm. Droplet deflections towards the right with a linear trajectory (constantθ) indicate that jumping droplets are positively charged and have achieved terminal velocity, respectively. (d) Experimental individual droplet charge (q) as a function of departing droplet radius (R) for uniform electric fieldsĒ=ΔV/d=1.31, 2.63 and 5.26 kV m−1. Droplet charging was independent of the applied electric field, indicating that induced charging effects are not responsible for the observed charging phenomena. Red dotted lines represent fits to the data for both regimes (R≲7 μm andR≳7 μm). Error bars denote the propagation of error associated with the high-speed camera resolution and the calculation of droplet size from terminal velocity obtained from high-speed image processing. The spread in the experimental data is expected because droplet coalescence can occur between two different size droplets as well as between more than two droplets (chamber vapour pressurePv=2,700±68 Pa,S≈1.04). Figure 3a,b shows top and side view schematics of the modified experimental setup, respectively (see Methods and Supplementary Fig. S5 ). Two polished copper plates (10 × 20 cm, Alloy 110, McMaster-Carr) were placed L =10±0.5 mm beneath the tube and spaced d =19±0.05 mm apart. The right plate ( Fig. 3b ) was grounded while the left plate was connected to the power supply. Control of the voltage bias and plate spacing allowed for accurate calculation of the magnitude and direction of the electric field ( E =Δ V / d ). A high-speed camera was mounted adjacent to the parallel plates to record the droplet motion between the plates. The camera was mounted ≈20 mm below the top of the plates to avoid non-parallel field edge effects and to allow droplets to reach terminal velocity before entering the field of view of the camera. Figure 3c shows long exposure time images (33 ms) of the droplet trajectory under applied electric fields of E=ΔV / d =1.31, 2.63 and 5.26 kV m −1 (right plate is grounded, see Supplementary Movies 11, 12 and 13 ) for the CuO superhydrophobic surface ( Fig. 1a ). The images show that (1) the droplet deflection θ was dependent on the electric field and (2) for each applied field, the deflection angle θ was constant, indicating that terminal velocity was reached. Droplets travelling at terminal velocity were analysed in terms of the forces in the x (horizontal) and y (vertical) directions. A charged droplet at terminal velocity experiences a force in the x direction of Σ F x =0=− F D sin θ + q E , and in the y direction of Σ F y =0= F D cos θ +( ρ v – ρ w ) V g , where F D is the drag force, θ is the angle between the droplet trajectory and the vertical, q is the charge on the droplet, ρ v and ρ w are the water vapour and liquid water densities, respectively, V is the droplet volume ( V =(4/3)π R 3 ) and g is the gravitational constant (see Supplementary Note 1 and Supplementary Fig. S6 ). The ratio of the two force components yields the trajectory equation q /[( ρ w – ρ v ) V ]=( g / E )tan θ . Figure 3: Experimental setup and images of droplet deflection. Schematic showing ( a ) top view and ( b ) side view of the experimental setup used to measure individual droplet charge. Two 10 × 20 cm polished parallel copper plates were placed L =10±0.5 mm beneath the tube and spaced d =19±0.05 mm apart. The plates were voltage biased relative to one another to create a uniform electric field. High-speed imaging of droplet motion inside the constant electric field beneath the tube sample allowed for the quantification of individual droplet charge for fields of Ē=ΔV / d =1.31, 2.63 and 5.26 kV m −1 . ( c ) Long exposure time images (33 ms) of droplet motion between the parallel plates at field strengths of Ē= 0, 2.63 and 5.26 kV/m (see Supplementary Movies 11, 12 and 13 ). Left side of the images is the positive plate and right side is the grounded plate. Scale bar, 4 mm. Droplet deflections towards the right with a linear trajectory (constant θ ) indicate that jumping droplets are positively charged and have achieved terminal velocity, respectively. ( d ) Experimental individual droplet charge ( q ) as a function of departing droplet radius ( R ) for uniform electric fields Ē=ΔV / d =1.31, 2.63 and 5.26 kV m −1 . Droplet charging was independent of the applied electric field, indicating that induced charging effects are not responsible for the observed charging phenomena. Red dotted lines represent fits to the data for both regimes ( R ≲ 7 μm and R ≳ 7 μm). Error bars denote the propagation of error associated with the high-speed camera resolution and the calculation of droplet size from terminal velocity obtained from high-speed image processing. The spread in the experimental data is expected because droplet coalescence can occur between two different size droplets as well as between more than two droplets (chamber vapour pressure P v =2,700±68 Pa, S ≈1.04). Full size image Figure 3d shows droplet charge as a function of droplet diameter on the CuO superhydrophobic surface for the three different field strengths ( E= 1.31, 2.63 and 5.26 kV m −1 ). The results show that there are two regimes: (1) for smaller radii ( R ≲ 7 μm), the droplet charge was independent of the surface area (~ R 0 ). This behaviour can be explained by examining the droplet growth before coalescence. Droplets growing on the superhydrophobic surface first nucleate within a structure unit cell, that is, area between the structures, eventually emerging from the unit cell to grow up and above the structures with a constant basal area [13] , [14] . Throughout this growth, the interfacial area between the structured surface and liquid droplet remains relatively constant as the droplet grows primarily by increasing its contact angle and forming a more spherical shape [14] , resulting in a constant electrostatic charge. (2) For large radii ( R ≳ 7 μm) the charge is droplet surface area-dependent (~ R 2 ) and is equal to q″ =7.8±3.6 μC m −2 . This dependency on surface area indicates that the charging mechanism of droplets is associated with the interfacial area between the condensing droplets and the hydrophobic surface beneath them when the growth phase enters the period of constant contact angle with increasing basal area expanding over the tips of the surface structures [13] . Furthermore, the results show that droplet charging was independent of the electric field strength, indicating that induced electrification or dielectrophoretic effects were not factors in the experiment. Droplet charging on different surfaces To further elucidate the potential mechanism of the droplet charging, we fabricated superhydrophobic surfaces spanning a range of length scales (~10 nm–1 μm) and materials including CuO, zinc oxide (ZnO) and silicon nanopillars (Si), shown in Fig. 4 (see Methods). To study the effects of the interfacial droplet–surface contact, we functionalized the surfaces with a variety of fluorinated and non-fluorinated hydrophobic coatings, including TFTS, thiol, Semblant Plasma Finish (SPF), P2i and stearic acid (see Fig. 4a–e , respectively, see Methods). Furthermore, to vary the effects of macroscale roughness and hierarchy, the CuO-nanostructured surfaces were created using smooth and rough Cu substrates having macroscale surface asperities on the order of ~10 nm and ~5 μm, respectively. Figure 5 shows the droplet charge q as a function of droplet radius R for all of the surfaces tested. 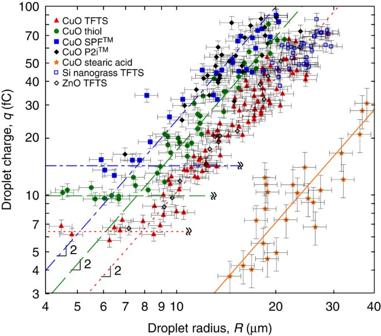Figure 5: Individual droplet charge as a function of droplet radius and condensing surface. Experimental individual droplet charge (q) as a function of departing droplet radius (R) for the structures shown inFig. 4for an electric fieldĒ=1.31 kV m−1(ΔV=25 V). Droplet charging is independent of the nanostructure material but dependent on the hydrophobic coating, which indicates charge separation at the interface due to the electric double layer formation. Dashed-green, dotted-red, dash-dot-blue and solid orange lines represent fits for the thiol, TFTS, SPF and P2i, and stearic acid coating data, respectively. It is important to note that, although OH−adsorption was present on all hydrophobic coatings tested, adsorption was approximately five times lower on the non-fluorinated coating (stearic acid) when compared with the fluorinated coatings, suggesting stronger affinity for OH−at water/fluoropolymer interfaces when compared with the water/hydrocarbon interface. Error bars denote the propagation of error associated with the high-speed camera resolution and the calculation of droplet size from terminal velocity obtained from high-speed image processing. The spread in the experimental data is expected because the droplet coalescence can occur between two different size droplets as well as between multiple droplets (chamber vapour pressurePv=2,700±68 Pa,S≈1.04). Surfaces with identical coatings, that is, CuO TFTS, ZnO TFTS, Si TFTS, showed identical charge trends ( q″ =7.8±3.6 μC m −2 ) irrespective of the surface structure or surface finish (see Supplementary Note 2 and Supplementary Figs S7 and S8 ). However, surfaces with differing coatings, that is, TFTS, thiol, Semblant Plasma Finish (SPF), P2i and stearic acid showed that charging was dependent on the hydrophobic coating ( q TFTS ″=7.8±3.6 μC m −2 , q thiol ″=12.6±2.6 μC m −2 , q SPF ″=17.0±4.1 μC m −2 , q P2i ″=17.2±3.9 μC m −2 , q stearic acid ″=1.39±0.9 μC m −2 ). 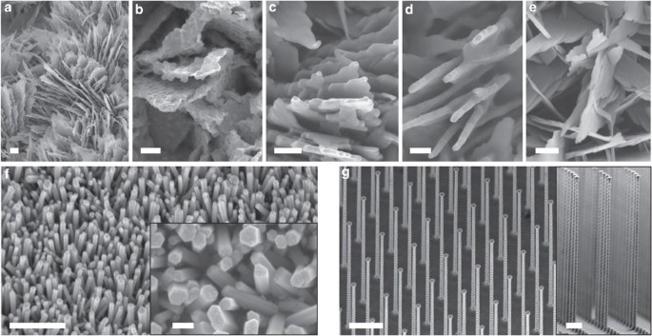This dependence of the coating indicates that the charging of the jumping droplets occurs at the solid–liquid interface, rather than after departing from the surface. Figure 4: Characterization of different hydrophobic coatings and micro/nanostructures. High-resolution field emission scanning electron micrographs of the tested surfaces including (a) CuO metal oxide coated with TFTS (scale bar, 200 nm), (b) CuO metal oxide coated with thiol (scale bar, 200 nm), (c) CuO metal oxide coated with SPF (scale bar, 200 nm), (d) CuO metal oxide coated with P2i (scale bar, 200 nm), (e) CuO metal oxide coated with stearic acid (scale bar, 200 nm), (f) ZnO metal oxide coated with TFTS, scale bar, 400 nm (inset: high-resolution image of the ZnO TFTS. scale bar, 60 nm), (g) silicon nanopillars coated with TFTS, scale bar, 2 μm (inset: high-resolution image of the Si nanopillar-TFTS. scale bar, 1 μm). All hydrophobic coatings were highly conformal and <60 nm in thickness, allowing for the CuO, ZnO and Si pillar shapes to be well preserved after coating. Figure 4: Characterization of different hydrophobic coatings and micro/nanostructures. High-resolution field emission scanning electron micrographs of the tested surfaces including ( a ) CuO metal oxide coated with TFTS (scale bar, 200 nm), ( b ) CuO metal oxide coated with thiol (scale bar, 200 nm), ( c ) CuO metal oxide coated with SPF (scale bar, 200 nm), ( d ) CuO metal oxide coated with P2i (scale bar, 200 nm), ( e ) CuO metal oxide coated with stearic acid (scale bar, 200 nm), ( f ) ZnO metal oxide coated with TFTS, scale bar, 400 nm (inset: high-resolution image of the ZnO TFTS. scale bar, 60 nm), ( g ) silicon nanopillars coated with TFTS, scale bar, 2 μm (inset: high-resolution image of the Si nanopillar-TFTS. scale bar, 1 μm). All hydrophobic coatings were highly conformal and <60 nm in thickness, allowing for the CuO, ZnO and Si pillar shapes to be well preserved after coating. Full size image Figure 5: Individual droplet charge as a function of droplet radius and condensing surface. Experimental individual droplet charge ( q ) as a function of departing droplet radius ( R ) for the structures shown in Fig. 4 for an electric field Ē =1.31 kV m −1 (Δ V =25 V). Droplet charging is independent of the nanostructure material but dependent on the hydrophobic coating, which indicates charge separation at the interface due to the electric double layer formation. Dashed-green, dotted-red, dash-dot-blue and solid orange lines represent fits for the thiol, TFTS, SPF and P2i, and stearic acid coating data, respectively. It is important to note that, although OH − adsorption was present on all hydrophobic coatings tested, adsorption was approximately five times lower on the non-fluorinated coating (stearic acid) when compared with the fluorinated coatings, suggesting stronger affinity for OH − at water/fluoropolymer interfaces when compared with the water/hydrocarbon interface. Error bars denote the propagation of error associated with the high-speed camera resolution and the calculation of droplet size from terminal velocity obtained from high-speed image processing. The spread in the experimental data is expected because the droplet coalescence can occur between two different size droplets as well as between multiple droplets (chamber vapour pressure P v =2,700±68 Pa, S ≈1.04). Full size image Based on our results, we propose a charge separation mechanism governed by the critical time scale associated with the droplet coalescence. It is well known that most hydrophobic coatings have a negative zeta potential [3] , [8] . In the presence of liquid water, these surfaces tend to adsorb negative charge and form an electric double layer in the fluid. Although the water used in these experiments is deionized, the dissociation of water molecules into their HO − and H + constituents continues in equilibrium [3] . As water droplets nucleate and grow on the superhydrophobic surface, OH − ions transport to the coating and preferentially adsorb to the surface, forming an electric double layer at the coating surface inside the nanostructure unit cell [6] . If the droplet is removed fast enough (coalescence and jumping), charge separation can occur, resulting in H + accumulation inside the jumping droplet. However, if the droplet is removed slowly, the motion of the contact line and subsequent accumulation of H + in the droplet will create a counter electric field, accelerating the desorption of the OH − ions and ensuring net neutrality of the removed droplet. To gain a better understanding of these dynamic processes, the time scales associated with each (coalescence, diffusion and electrophoresis) are considered. For water droplets of radii R ≳ 2 μm, coalescence is governed by an inertially limited viscous regime at low neck radii ( R min / R ≤ Oh , where R min is the radius of the neck connecting the two coalescing droplets and Oh is the characteristic droplet Ohnesorge number defined by Oh = μ /( ρ w σ R ) 1/2 ) and by an inertial regime at larger neck radii ( R min / R > Oh ) [44] . Due to the relatively low Ohnesorge number, Oh ≈0.02–0.1 (for the droplet range analysed here, 2 μm< R <40 μm), the majority of droplet coalescence (>90% for R =2 μm) occurs in the inertial regime [44] , where the time scale is governed by a capillary inertial scaling [45] , [46] , [47] , τ c ~( ρ w R 3 / σ ) 1/2 . Furthermore, the coalescence dynamics of the inertially limited viscous regime are faster than the inertial regime [44] , such that τ c is an over-estimate (see Supplementary Note 3 ) and an appropriate upper bound for the coalescence time scale. The time scales for charge transport from the hydrophobic coating to the droplet bulk can be characterized by two separate mechanisms, diffusion of the desorbed ion through the liquid residing in the structure [48] τ d ~[ h /(2 D H+ 1/2 )] 2 and electrophoresis of the desorbed ion due to the formation of the counter electric field [49] τ e ~ h /[ Ē* μ e,H+ )], where h is the characteristic structure height, D H+ is the diffusivity of the H + ion, μ e,H+ is the combined electrophoretic and electroosmotic mobility of the H + ion and E* is the magnitude of the counter electric field (approximated as E* ≈ ζ / h , where ζ is the hydrophobic coating zeta potential). In addition to H + ions, H 3 O + and OH − ions were analysed, however, H + is discussed herein due to its higher diffusivity and mobility, allowing for a conservative estimate of the critical time scales (for analysis of H 3 O + and OH − , see Supplementary Note 3 and Supplementary Fig. S9 ). As mentioned previously, if the time scale of the coalescence process is fast enough, insufficient time is available for OH − desorption and subsequent transport to the droplet bulk before it jumps. Comparing the characteristic time scales shows that τ c / τ d <<1 and τ c / τ e <<1 for the entire range of measured droplet charge and ion type (see Supplementary Fig. S9 ), suggesting that, although a counter electric field develops at the rapidly moving contact line during coalescence, the time needed for OH − desorption and transport to the droplet bulk is not sufficient, leaving OH − adsorbed to the surface while resulting in a positively charged jumping droplet. The electrical ( τ e ) and hydrodynamic ( τ d ) time scales defined above have been commonly studied for coupled hydrodynamic-electrical phenomena, such as charged liquid jets [50] , to differentiate the phenomena of charge relaxation and charge separation [50] , [51] , [52] . Due to the similar magnitudes of the electrical and hydrodynamic time scales ( τ e / τ d =(4 D H+ )/( ζ μ e,H+ )≈1.35), the time scales can be approximated as τ e ≈ τ d = ε i / K , where ε i is the permittivity of liquid water and K is the combined ionic (or electrical) conductivity of pure water [51] . In this case, τ e ≈ τ d = ε i / K ≈130 μs, which agrees well with our calculated values of 165 and 125 μs for H + ions. To further support the proposed charge separation mechanism, we determined the effective zeta potential of the charged surfaces with our measurements. The zeta potential of the thiol, TFTS, SPF, P2i and stearic acid coatings was determined to be ζ thiol ≈−84 mV, ζ TFTS ≈−56 mV, ζ SPF ≈ ζ P2i ≈−121 mV, ζ stearic acid ≈−19 mV, respectively (see Supplementary Note 4 ). These values are reasonable estimates considering most fluoropolymer coatings have typical zeta potentials in the range of −25 to −85 mV (ref. 3 ). Furthermore, to experimentally verify the proposed charge separation mechanism, high-speed video of departed droplet return towards a horizontally oriented nanostructured CuO surface was analysed. Analysis of the video showed droplets ( R ≈9±4.7 μm, initially travelling at a terminal velocity downwards due to gravity) accelerating towards the surface once reaching a critical gap distance δ ≈250 μm between the droplet and the surface (see Supplementary Movie 14 and Supplementary Fig. S1 ). The observed acceleration of droplets is in contrast to previous studies of electrically neutral droplets falling towards a wall, which show that the drag force on a droplet increases when the gap between the droplet and wall vanishes at constant velocity, resulting in droplet deceleration [53] . The observed acceleration occurs due to the charge separation and attractive electrostatic force between the positively charged droplet and the negatively charged CuO hydrophobic wall. This result further supports the proposed charge separation mechanism. In the future, it would be interesting to examine the droplet charging phenomena of larger coalescence-induced jumping droplets ( R >100 μm) to gain a better understanding of droplet charging dynamics as the coalescence time scale ( τ c ) approaches the characteristic times τ e and τ d ( τ c ~ τ e ). It is expected that as τ c ~ τ e , deviation from the ~ R 2 -dependent droplet charging phenomena would occur and smaller droplet charging would be observed due to sufficient time for charge re-combination and smaller charge separation. Studying the effect of similar time scales on such large droplets ( R >100 μm) was not possible here due to the large nucleation densities realized during the experiments. This work offers new opportunities for a wide variety of possible applications such as the use of external electric fields to control the jumping frequency from the surface to increase condensation heat transfer [13] , enhance anti-icing [24] , improve self-cleaning performance [12] and enhance thermal diode efficiency [22] . In addition, by providing a relative measure of the charge adsorption, a new metrology can be developed to characterize the electrokinetic properties, such as the zeta potential, of hydrophobic materials and coatings on large-scale surfaces [54] . Furthermore, the identified electric double layer charge separation [41] and droplet charging can be used for atmospheric energy harvesting and electric power generation, where charged droplets jump between superhydrophobic and hydrophilic surfaces to create an electrical potential. Surface fabrication To create the CuO nanostructures ( Fig. 1a ), commercially available oxygen-free Cu tubes were used (99.9% purity) with outer diameters, D OD =6.35 mm, inner diameters, D ID =3.56 mm, and lengths, L =131 mm, as the test samples for the experiments. Each Cu tube was cleaned in an ultrasonic bath with acetone for 10 min and rinsed with ethanol, isopropyl alcohol and deionized (DI) water. The tubes were then dipped into a 2.0-M hydrochloric acid solution for 10 min to remove the native oxide film on the surface, then triple-rinsed with DI water and dried with clean nitrogen gas. Nanostructured CuO films were formed by immersing the cleaned tubes (with ends capped) into a hot (96±3 °C) alkaline solution composed of NaClO 2 , NaOH, Na 3 PO 4 ·12H 2 O and DI water (3.75: 5: 10: 100 wt%) [55] . During the oxidation process, a thin (≈300 nm) Cu 2 O layer was formed that then re-oxidized to form sharp, knife-like CuO oxide structures with heights of h ≈1 μm, a solid fraction φ ≈0.023 and a roughness factor r ≈10. The ZnO nanowires ( Fig. 4f ) with diameters of d ≈40 nm, heights h ≈350 nm and centre-to-centre spacings of l ~100 nm (solid fraction φ = πd 2 /4 l 2 ≈0.056 and roughness factor r =1+ πdh / l 2 ≈2.95) were synthesized in solution according to the procedures of Pacholski, Kornowski and Weller [56] . To synthesize ZnO seed crystals, 0.01 M of zinc acetate dihydrate (Sigma-Aldrich, ACS reagent, ≥99.0%) and 0.03 M of sodium hydroxide (Sigma-Aldrich, ACS reagent, ≥98.0%) in methanol were mixed and stirred at 60 °C for 2 h. The resulting solution was used to create ZnO seed crystals onto desired substrates by drop-coating, followed by rinsing with methanol and blow-drying with a weak stream of nitrogen. This drop-coating process was repeated five times. The ZnO seed crystals were then bonded by annealing the substrate at 350 °C for 20 min in air. Hydrothermal growth of the ZnO nanowires was achieved by placing the substrate in an aqueous solution containing 0.025 M of zinc nitrate (purum pro analysis, crystallized, ≥99.0%) and 0.025 M of hexamethylenetetramine (Sigma-Aldrich, ACS reagent, ≥99.0%) at 90 °C for 2 h. Silicon nanopillar surfaces ( Fig. 4g ) with diameters of d =200 nm, heights of h =10 μm and centre-to-centre spacings of l =2 μm (solid fraction φ = πd 2 /4 l 2 =0.0079 and roughness factor r =1+ πdh ′/ l 2 =3.47) were fabricated using projection lithography and deep reactive ion etching. Surface functionalization TFTS was deposited from the vapour phase ( Fig. 4a ). Before silane deposition, each tube was oxygen plasma cleaned for 2 h to remove organic contaminants on the surface. Once clean, the tube samples were immediately placed in a vacuum desiccator (06514-10, Cole Parmer) with a small amount of liquid silane. The desiccator was evacuated by a roughing pump for 2 min to a minimum pressure of ≈2 kPa. A valve was then closed to isolate the pump from the desiccator and the sample was held in vacuum (≈2 kPa) for another 7 min. The silanated tubes were then rinsed in ethanol and DI water and dried in a clean nitrogen stream. Thiol functionalization ( Fig. 4b ) was achieved by first sputtering a ≈30-nm-thick coating of Au onto the CuO nanostructures. The samples were then solvent rinsed, dried and plasma cleaned before immersion into a 1-mM solution of 1H, 1H, 2H, 2H-perfluorodecanethiol (Sigma-Aldrich) in ethanol for 1 h. Goniometric measurements (MCA-3, Kyowa Interface Science) of ≈100 nl droplets on a smooth thiolated surface showed advancing and receding contact angles of θ a =121.1°±2.2° and θ r =106.3°±2.4°, respectively. The SPF fluoropolymer coating ( Fig. 4c ) was achieved with a plasma polymer process. The CuO sample was loaded into a vacuum chamber. Once basic vacuum was achieved, a precursor gas was pumped into the chamber and a radio frequency voltage was generated to convert the gas into plasma. This process involves the stripping of electrons from the precursor molecule, as well as fragmentation of the molecule into neutral, charged and radical species. These reactive species reassembled on the surface of the sample in the chamber to create a highly conformal (≈40-nm thick) hydrophobic fluoropolymer coating. Goniometric measurements (MCA-3, Kyowa Interface Science) of ≈100 nl droplets on a smooth SPF-coated silicon wafer surface showed advancing and receding contact angles of θ a =114.8°±2.6° and θ r =103.0°±3.2°, respectively. The P2i hydrophobic coating ( Fig. 4d ) was achieved with plasma-enhanced vapour deposition. The process occurs under low pressure within a vacuum chamber at room temperature. The coating is introduced as a vapour and ionized. This process allows for the development of a highly conformal (≈30-nm thick) polymer layer, which forms a covalent bond with the CuO surface, making it extremely durable. Goniometric measurements (MCA-3, Kyowa Interface Science) of ≈100 nl droplets on a smooth P2i-coated silicon wafer surface showed advancing and receding contact angles of θ a =124.3°±3.1° and θ r =112.6°±2.8°, respectively. Stearic acid ( n -octadecanoic acid, Sigma-Aldrich, Fig. 4e ) was bonded to the surface following a procedure adapted from work by Wu et al [57] . Samples were solvent rinsed and plasma cleaned for 1 h, then immersed in a 0.1-mM solution of stearic acid in n-hexane (≥99%, Sigma-Aldrich) at room temperature. After 48 h, the samples were removed from solution, rinsed in acetone and dried in a clean nitrogen stream. Goniometric measurements (MCA-3, Kyowa Interface Science) of ≈100 nl droplets on a smooth stearic acid-coated copper surface showed advancing and receding contact angles of θ a =109.2°±4.8° and θ r =88.1°±5.1°, respectively. Surface characterization Advancing and receding contact angles for all samples were measured and analysed using a microgoniometer (MCA-3, Kyowa Interface Science, Japan). Field emission electron microscopy was performed on a Zeiss Ultra Plus FESEM (Carl Zeiss GMBH) at an imaging voltage of 3 kV. Experimental apparatus The custom environmental chamber used for this work (Kurt J. Lesker Company) consists of a stainless steel frame with a door (sealed with a rubber gasket), two viewing windows and apertures for various components ( Supplementary Fig. S2 ). Resistive heater lines were wrapped around the exterior of the chamber walls to prevent condensation at the inside walls and then insulated on the exterior walls. The output power of the resistive heater lines was controlled by a voltage regulator (Variac). Two insulated stainless steel water flow lines (Swagelok) were fed into the chamber via a KF flange port (Kurt J. Lesker Company) to supply cooling water to the chamber from a large capacity chiller (System III, Neslab). A flow meter (5 LPM MAX, Alicat) having an accuracy of ±2% was integrated along the water inflow line. A secondary stainless steel tube line was fed into the chamber via a KF adaptor port that served as the flow line for the incoming water vapour supplied from a heated steel water reservoir. The vapour line was wrapped with a rope heater (60 W, Omega) and controlled by a power supply (Agilent). The vapour reservoir was wrapped with another independently controlled rope heater (120 W, Omega) and insulated to limit heat losses to the environment. The access tubes were welded to the vapour reservoir, each with independently controlled valves. The first valve (Diaphragm Type, Swagelok), connecting the bottom of the reservoir to the ambient, was used to fill the reservoir with water. The second valve (BK-60, Swagelok), connecting the top of the reservoir to the inside of the chamber, provided a path for vapour inflow. K-type thermocouples were located along the length of the water vapour reservoir to monitor temperature. A bellows valve (Kurt J. Lesker Company) was attached to the chamber to serve as a leak port between the ambient and inside of the chamber. To monitor temperatures within the chamber, K-type thermocouple bundles were connected through the chamber apertures via a thermocouple feed through (Kurt J. Lesker Company). To provide electrical connections inside the chamber for light-emitting diode lighting and electric field generation, insulated copper electrical wires were connected through the chamber apertures via an electrical feed through (Kurt J. Lesker Company). A pressure transducer (925 Micro Pirani, MKS) was attached to monitor pressure within the chamber. The thermocouple bundles and the pressure transducer were both electrically connected to an analogue input source (RAQ DAQ, National Instruments), which was interfaced to a computer for data recording. A second bellows valve (Kurt J. Lesker Company) was integrated onto the chamber for the vacuum pump, which brought down the chamber to vacuum conditions before vapour filling. A liquid nitrogen cold trap was incorporated along the line from the chamber to the vacuum, which served to remove any moisture from the pump-down process and ultimately assist in yielding higher quality vacuum conditions. A tertiary bellows valve (Kurt J. Lesker Company) was integrated on a T fitting between the vacuum pump and liquid nitrogen reservoir to connect the vacuum line to the ambient to release the vacuum line to ambient conditions once pump down was achieved. To visually record data, a high-speed camera (Phantom v7.1, Vision Research) was placed in line with the 5′′ viewing windows on the chamber. In addition, a digital SLR camera (Cannon) was interchangeable with the high-speed camera to obtain colour images. The schematic of the exterior of the environmental setup is depicted in Supplementary Fig. S2a . Images of the front and rear of the experimental setup are shown in Supplementary Fig. S2b,c respectively. To run the test samples inside the chamber, the stainless steel bellows tube lines (1/4′′, Swagelok) were connected to the external water flow lines ( Supplementary Fig. S2c ). T-connection adaptors (Swagelok) with bore through Ultra-Torr fittings (Swagelok) were used to adapt K-type thermocouple probes (Omega) at the water inlet and outlet. Before experimentation, the thermocouple probes were calibrated using a high-precision temperature-controlled bath (Lauda Brinkman, LP.) to an accuracy of ±0.1 K. The test samples, 6.35 mm outer diameter tubes with different surface treatments, were connected via a Swagelok compression fitting onto the T-connection. Chilled water flows through the inlet bellows tube, along the inside of the tube sample and through the outlet. Two supports were used to hold the sample and the entire configuration in place. Two separate pieces of insulation were embedded with K-type thermocouple leads and used for wet bulb temperature measurement during experimental runs. A third thermocouple was placed beside the sample to measure the reference temperature inside the chamber ( Supplementary Fig. S3 ). Condensation experimental procedure For each experimental trial, a set of strict procedures were followed to ensure consistency throughout the experiments. The first step of the process was to turn on the voltage regulator to heat up the environmental chamber walls, which prevented condensation on the chamber walls. Simultaneously, the water vapour reservoir was filled with ~3.5 l of DI water (99% full) using a syringe through the vapour release valve. After opening the vapour inflow valve and closing the vapour release valve, the rope heater around the water vapour reservoir was turned on with the heater controller set to maximum output (120 W). Then the rope heater connected to the vapour inflow valve was turned on. The temperature of the water reservoir was monitored with the installed thermocouples; the temperature at the top of the reservoir was higher than that of the middle/bottom of the reservoir due to the water thermal-mass present at the middle/bottom section. Hence, we ensured that the regions of the water reservoir of higher thermal capacity were brought to a sufficiently high temperature for boiling. During the boiling process, aluminium foil was placed on the bottom surface of the inner chamber to collect any of the water leaving the vapour inflow line. Once boiling was achieved and all thermocouples on the reservoir were >95 °C for at least 10 min, the vapour inflow valve was closed. The excess water that spilled inside the chamber during de-gassing of the reservoir was removed. To install the samples onto the rig ( Supplementary Fig. S3 ), the Swagelok female adaptors at the ends of the tube samples were connected to the 90° male elbow connecters on the rig. Before installing the entire sample setup in the chamber, all adaptors/connecters were tightened to ensure that there were no leaks that could affect vacuum performance. The setup was then placed on top of the steel supports and the bellows tubes (for the water inflow/outflow) were connected to the water lines. Then, the insulating wet bulb wick was placed near the sample and in contact with the bottom surface of the chamber. The next step was to begin the vacuum pump-down procedure. Initially, the liquid nitrogen cold trap was filled to about half capacity. The ambient exposed valves connecting the chamber and the vacuum pump were both closed and the valve connected to the liquid nitrogen cold trap was opened. The vacuum pump was then turned on, initiating the pump-down process. The pressure inside the chamber was monitored during the pump-down process. This process took ~1 h to achieve the target vacuum conditions (0.5 Pa< P <1 Pa). The experimental operating pressure of non-condensable was set to be a maximum of 0.25% of the operating pressure. Non-condensable gas content of above 0.5% (pressure) was shown to significantly degrade performance during dropwise condensation. In our experiments, extreme care was taken to properly de-gas the vacuum chamber and water vapour reservoir prior to experimental testing. In addition, the chamber leak rate was characterized before each run to estimate the maximum time available for acquiring high-fidelity data with non-condensable content of <0.25%. The setup of the water flow loop is described as follows. The Neslab water pump reservoir was filled and turned on to a flow rate of 5 l min −1 (0<Δ T LMTD <15 K). The flow rate was monitored with the flow meter integrated in the inflow water line. To bring the chilled water into the flow loop and to the tube sample, the external chilled water lines were opened. Before beginning experiments, the high-speed camera was turned on for visual recording of the sample during condensation. Afterwards, the rope heater around the water reservoir was turned off and the vapour inflow valve was slowly turned open until the operating pressure was reached. Steady-state conditions were typically reached after 2 min of full operation. Charge polarity experimental procedure To study the effect of droplet charging, the experimental setup was modified to include an electrode placed beneath the CuO-nanostructured tube ( Supplementary Fig. S4 ). The electrode (red insulated wire) was connected to the insulated copper electrical feed through and brought in close proximity (<1 cm) to the tube via an insulated copper holder made from a strip of copper sheet. To electrically insulate the holder, a piece of insulation was placed beneath it ( Supplementary Fig. S4a ). The electrode was energized by an external 600 V DC power supply (Agilent Technologies, N5752A). The negative terminal of the power supply was grounded to the tube. The terminals could be reversed externally to study the polarity of the droplet charge by reversing the direction of the established electric field between the electrode and grounded tube. Supplementary Fig. S4c,d shows typical views from the side viewport of the tube–electrode setup before and after condensation initiates (Δ V =0 V), respectively. To monitor the local temperature close to the electrode, a K-type thermocouple was placed in close proximity ( Supplementary Fig. S4c,d ). Charge measurement experimental procedure To study the magnitude of the charge imparted on the droplet (in addition to verifying the polarity), a Millikan [1] -inspired parallel plate setup was used to establish a uniform electric field. The previously discussed wire electrode setup was advantageous in providing a simple measure of charge polarity; however, it was difficult to utilize for calculating the magnitude of the charge. The difficulty was related to potential charge accumulation on the hydrophobic coating [6] , [58] , making it difficult to determine an accurate electric field magnitude. In addition, the non-uniform electric field established between the tube and electrode added increased complexity to the charge calculation. Furthermore, the non-uniform electric field had the potential to create a dielectrophoretic force component on the jumping droplets [54] , creating additional difficulty for the determination of droplet charge. To accurately obtain the magnitude of the charge on the droplets, we used a uniform electric field. Two 10 × 20 cm polished copper plates (McMaster) were arranged in a parallel configuration ( Supplementary Fig. S5a ) and placed beneath the tube sample ( Supplementary Fig. S5b ). One plate was connected to ground (right plate when viewed from the front viewport), while the other was energized by the external DC power supply (left plate when viewed from the front view port, Supplementary Fig. S5c,d ). The ground plate was also connected to the tube (red wire, Supplementary Fig. S5c ) to ensure an accurate potential measurement. The bottom sides of the plates were masked with Teflon tape, providing electrical insulation from the chamber walls. The light-emitting diode light ( Supplementary Fig. S5b ) was placed behind the plates and shining between them towards the view port. Once condensation initiated, droplets jumping from the surface were captured between the parallel plates, reaching terminal velocity in the process and allowing for the trajectory to be analysed. The high-speed and SLR cameras were used to image the droplet motion between the plates. The focal plane was set to lie beneath the tube where droplet motion was frequent. How to cite this article: Miljkovic, N. et al. Electrostatic charging of jumping droplets. Nat. Commun. 4:2517 doi: 10.1038/ncomms3517 (2013).